Pioneer glutamatergic cells develop into a morpho-functionally distinct population in the juvenile CA3 hippocampus The developing CA3 hippocampus is comprised by highly connected hub neurons that are particularly effective in achieving network synchronization. Functional hub neurons were shown to be exclusively GABAergic, suggesting that the contribution of glutamatergic neurons to physiological synchronization processes at early postnatal stages is minimal. However, without fast GABAergic transmission, a different situation may prevail. In the adult CA3, blocking fast GABAergic transmission induces the generation of network bursts that can be triggered by the stimulation of single pyramidal neurons. Here we revisit the network function of CA3 glutamatergic neurons from a developmental viewpoint, without fast GABAergic transmission. We uncover a sub-population of early-generated glutamatergic neurons that impacts network dynamics when stimulated in the juvenile hippocampus. Additionally, this population displays characteristic morpho-physiological features in the juvenile and adult hippocampus. Therefore, the apparently homogeneous glutamatergic cell population likely displays a morpho-functional diversity rooted in temporal embryonic origins. Synchronized discharges of cell populations are a characteristic feature of epileptic networks, as well as a hallmark of developing neuronal structures. Such network dynamics are highly dependent on the connectivity between various types of neurons. At early postnatal stages, the developing hippocampus displays spontaneous, synapse-driven network synchronizations in the form of giant depolarizing potentials (GDPs) [1] . We have previously shown that GDPs are dependent on superconnected GABAergic hub neurons for their generation, and that stimulating a single hub cell could affect GDPs in the CA3 region of mouse hippocampal slices [2] . Despite the profound contribution of GABAergic neurons to signalling, the majority of neurons contributing to the CA3 hippocampal network are pyramidal glutamatergic cells. Still, glutamatergic neurons could not impact GDPs occurrence when stimulated [2] . This demonstrates that despite their large numbers, the contribution of single glutamatergic neurons to physiological synchronization processes in the immature postnatal hippocampus is minimal. In the adult hippocampus, blocking the fast inhibitory GABAergic drive generates network bursts that are thought to mimic epileptic conditions. In these artificial conditions, Miles and Wong [3] have shown that stimulating a single CA3 pyramidal neuron in hippocampal slices from the adult guinea pig triggers network synchronization. Spontaneous firing in CA3a cells preceded population bursts in a larger proportion than in other regions while evoked firing in these cells more reliably induced an increase in multiunit activity [4] . Last, CA3a glutamatergic cells displayed distinct morpho-physiological properties including a greater excitability, as well as enhanced synaptic connectivity [5] . Therefore, a sub-population of glutamatergic neurons bears the potential to entrain large networks without the contribution of GABAergic signals. This population was proposed to act as ‘pacemaker’ cells [5] . Here, we investigated whether, already at early developmental stages, glutamatergic neurons could trigger comparable network bursts without the contribution of GABAergic transmission. Given that embryonic origin was recently shown to predict GABAergic hub cell fate [6] , we investigated whether glutamatergic neurons endowed with the capability to trigger network bursts also originate from specific embryonic time points. To address the above issues, we studied the postnatal maturation of the network function of single CA3 pyramidal neurons when artificially blocking fast GABAergic transmission. We used multibeam calcium imaging to analyse the sequential activation of CA3 neurons. Immature (P7) and juvenile (P14 onwards) postnatal stages were compared. Targeted patch-clamp recordings were performed to assess the network power of individual neurons as a function of their temporal recruitment and to determine their morpho-physiological properties. Inducible genetic fate mapping approaches were used to compare the network involvement of early and late generated glutamatergic neurons (EGNs and LGNs). We show that neurons are sequentially recruited into network bursts according to their temporal embryonic origin, with EGNs being recruited before LGNs. Moreover, small assemblies of EGNs can trigger network bursts when stimulated at P7, while individual ones can generate similar bursts at juvenile stages. In contrast, stimulating LGNs has no impact on network dynamics. Additionally, in the adult hippocampus, EGNs segregate in the deeper parts of CA3a/b and display a combination of morpho-physiological features that should enable them to be early activated and influence the activity of other neurons. Therefore, the ultimate morpho-physiological and functional diversity of CA3 glutamatergic neurons seems to originate from their date of birth. CA3 dynamics in the absence of GABA A -R transmission In order to measure the development of the contribution of single CA3 pyramidal neurons to network function one needs to be able to simultaneously control the activity of individual neurons, while measuring network dynamics. In the developing hippocampus (P7), this can be achieved using two-photon calcium imaging in combination with electrophysiological recordings [2] . Unfortunately, at juvenile and adult stages only a small fraction of CA3 neurons can be loaded with acetoxymethyl (AM) ester fluorescent dyes in slices [7] . Therefore, the network involvement of single neurons was tested by combining single-cell recordings with: (1) multi-neuron calcium imaging at P7; (2) extracellular field potential recordings from P14 onwards. At P7, there is a strict correlation between the events measured using both approaches ( n =5 slices, Supplementary Fig. S1 ). Cells that function in synchronizing neuronal activity are expected to be activated at the onset of spontaneous network events [2] , [5] . In order to identify such cells, we first analysed the sequences of neuronal activation occurring spontaneously in the CA3 region, in contexts where fast GABAergic signalling is artificially removed through the application of GABA A -R antagonists. To sample the widest hippocampal area possible, we used a low magnification objective ( × 10, Fig. 1 ) at P7, and multiple field potential recordings or Microelectrode Arrays (MEAs, Fig. 2 ) at P14 and onwards. At P7, even though GABAergic transmission is still excitatory in many developing neurons and as previously described [1] , [8] , GABA A -Rs blockade in thick slices (see Methods and Supplementary Fig. S2 ) triggers spontaneous network bursts occurring on average every 13.7±2.2 s and involving 71±3% of the imaged cells ( n =18 movies). Similar event frequencies were observed at P14–20. Later (P45–120), network bursts are sparse and irregular, a condition which unfortunately precludes analysing the impact of single-cell stimulation on event frequency with statistical relevance ( Supplementary Fig. S3 ). 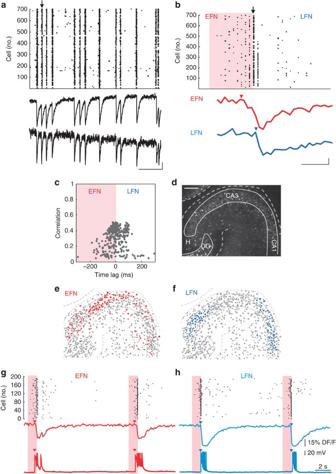Figure 1: Spatio-temporal network dynamics in the absence of fast GABAergic transmission in the developing CA3 region. (a) Top: Rasterplot of the calcium event onsets as a function of time for every neuron imaged in the presence of bicuculline (10 μM) in a P7 mouse hippocampal slice loaded with Fura-2AM and recorded with two-photon multibeam excitation at X10 magnification. Bottom traces show two representative calcium fluorescence traces from two cells in the network. Scale bar:xaxis: 30 s,yaxis: 10% DF/F. (b) Top: Rasterplot showing the temporal recruitment of the neurons involved in a representative network burst (marked by an arrow in (a)). Orange area indicates the time of activation of EFN while white area indicates that of LFN. Arrow indicates the peak of maximum cell coactivation. Two examples of calcium fluorescence changes occurring in an EFN (red) and a LFN (blue) during that event are illustrated below. Scale bar:xaxis: 1 s,yaxis: 10% DF/F. (c) Time-lag correlation graph plotting for each imaged neuron (729 neurons) the average correlation and average time of activation relative to all other cells for all network bursts within a recording session (12 events). The peak of maximum cell coactivation (arrow inb) was used as the zero time reference. (d) Two-photon calcium fluorescence image of the recorded network. Scale bar: 100 μm. (e) Contour plot of the cells imaged in (b). Red filled contours indicate EFNs. (f) Same as (e) with LFNs filled in blue. (g,h) Simultaneous calcium imaging and patch-clamp recording of EFNs (red,g) and LFNs (blue,h) in the CA3 region of a P7 mouse slice. Top rasterplots indicate the fraction of active cells as a function of time. In both cases, two network bursts were recorded. Arrows indicate the activation onsets of the EFN (red) and LFN (blue). Middle traces illustrate the calcium fluorescence changes in EFNs and LFNs and bottom traces show the simultaneous membrane potential changes recorded in current-clamp mode at resting membrane potential (I~0 pA) in the EFN (red) and LFN (blue). Figure 1: Spatio-temporal network dynamics in the absence of fast GABAergic transmission in the developing CA3 region. ( a ) Top: Rasterplot of the calcium event onsets as a function of time for every neuron imaged in the presence of bicuculline (10 μM) in a P7 mouse hippocampal slice loaded with Fura-2AM and recorded with two-photon multibeam excitation at X10 magnification. Bottom traces show two representative calcium fluorescence traces from two cells in the network. Scale bar: x axis: 30 s, y axis: 10% DF/F. ( b ) Top: Rasterplot showing the temporal recruitment of the neurons involved in a representative network burst (marked by an arrow in ( a )). Orange area indicates the time of activation of EFN while white area indicates that of LFN. Arrow indicates the peak of maximum cell coactivation. Two examples of calcium fluorescence changes occurring in an EFN (red) and a LFN (blue) during that event are illustrated below. Scale bar: x axis: 1 s, y axis: 10% DF/F. ( c ) Time-lag correlation graph plotting for each imaged neuron (729 neurons) the average correlation and average time of activation relative to all other cells for all network bursts within a recording session (12 events). The peak of maximum cell coactivation (arrow in b ) was used as the zero time reference. ( d ) Two-photon calcium fluorescence image of the recorded network. Scale bar: 100 μm. ( e ) Contour plot of the cells imaged in ( b ). Red filled contours indicate EFNs. ( f ) Same as ( e ) with LFNs filled in blue. ( g , h ) Simultaneous calcium imaging and patch-clamp recording of EFNs (red, g ) and LFNs (blue, h ) in the CA3 region of a P7 mouse slice. Top rasterplots indicate the fraction of active cells as a function of time. In both cases, two network bursts were recorded. Arrows indicate the activation onsets of the EFN (red) and LFN (blue). Middle traces illustrate the calcium fluorescence changes in EFNs and LFNs and bottom traces show the simultaneous membrane potential changes recorded in current-clamp mode at resting membrane potential (I~0 pA) in the EFN (red) and LFN (blue). 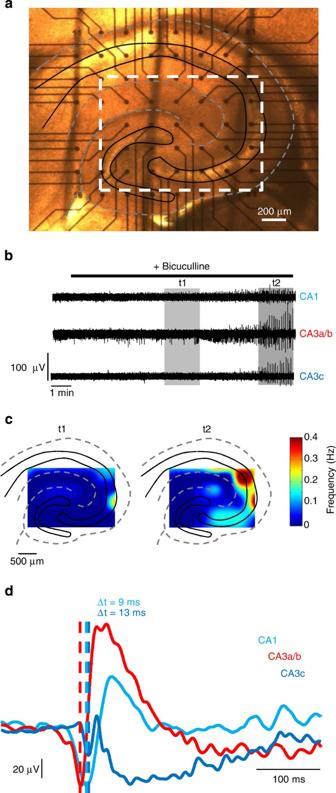Figure 2: Spatio-temporal network dynamics in the absence of fast GABAergic transmission in the juvenile CA3 region. (a) Photomicrograph from a P15 mouse hippocampal slice recorded with a MEA. Dashed rectangle indicates region of interest. (b) Simultaneous extracellular recordings of multiunit activity from electrodes localized at the border of CA3a/CA1 regions (top), in CA3a/b (middle) and in the CA3c region (bottom). (c) Colour coded spatial representation of the regions activated at the two successive time windows indicated by grey rectangles inb. Red indicates the most active regions while areas in blue are inactive. (d) Simultaneous triple field potential recordings of a single network burst recorded at three different locations (CA1 (light blue), CA3a/b (red) and in CA3c (dark blue)). In the absence of GABAA-R-mediated transmission, network bursts are first generated in the CA3a/b region. Full size image Figure 2: Spatio-temporal network dynamics in the absence of fast GABAergic transmission in the juvenile CA3 region. ( a ) Photomicrograph from a P15 mouse hippocampal slice recorded with a MEA. Dashed rectangle indicates region of interest. ( b ) Simultaneous extracellular recordings of multiunit activity from electrodes localized at the border of CA3a/CA1 regions (top), in CA3a/b (middle) and in the CA3c region (bottom). ( c ) Colour coded spatial representation of the regions activated at the two successive time windows indicated by grey rectangles in b . Red indicates the most active regions while areas in blue are inactive. ( d ) Simultaneous triple field potential recordings of a single network burst recorded at three different locations (CA1 (light blue), CA3a/b (red) and in CA3c (dark blue)). In the absence of GABA A -R-mediated transmission, network bursts are first generated in the CA3a/b region. Full size image At P7, the build-up of activity during network bursts lasted on average 575±41 milliseconds ( Fig. 1b , n =8 slices). To reveal if a characteristic pattern of cells was recruited in the build-up period, we compared between different network bursts, the pattern of cells activated within 500 ms before the peak of synchrony. Similarity between cell activation patterns was measured using cluster analysis and compared with reshuffled data for statistical significance (see Methods and ref. 2 ). We observed that network bursts were characterized by a stereotypical sequence of neuronal activation that accounted for most of the events occurring within the recording period (77±6% events, n =5 slices, Fig. 1a–f ). This indicates that the sequences of neuronal activation in the absence of fast GABAergic transmission are almost invariable. In contrast, the network bursts occurring in physiological conditions display more variability as only one-third of GDPs occurring within a recording period presented similar dynamics [2] . Based on the cross-correlation between the firing of cell pairs, for each neuron, we estimated the average correlation and time lag of activation relative to all other cells ( Fig. 1c , Methods and [2] ). These time-lag correlation graphs presented a bimodal distribution ( Fig. 1c ) with neurons clustered on the upper left region of the graph being reliably activated during the build-up of most network bursts (early firing neurons, (EFNs) see Methods , Fig. 1c ) while neurons on the right were activated after (late firing neurons (LFNs) Fig. 1c ). In some recordings we could compare the time of activation of neurons before and after adding the GABA A -R blocker. Interestingly, we found that a large majority (88%, n =4 slices) of the cells were detected as early firing both in control and drug conditions (not shown). In the low magnification recordings, we found that EFNs preferentially distributed in the CA3a/b region while LFNs were located in peripheral regions (CA1 and CA3c, Fig. 1d–f ). Similarly, at P14 and onwards, CA3a/b was found to be a preferential initiation site ( Fig. 2 ). In fact, after bicuculline was washed in, MEA recordings of single unit activity indicated that synchronization first appeared in CA3a/b, sequentially followed by CA1 and CA3c with a delay of 9.8±8.4 s and 18.4±9.2 s, respectively ( n =5 slices, Fig. 2b ). In addition, once stable conditions of burst generation were reached, field potential recordings indicated that network bursts were initiated on average 4.5±1.1 ms and 7.5±1.2 ms in CA3a/b before CA1 and CA3c, respectively ( n =5 slices, Fig. 2d ). We conclude that at all postnatal stages CA3a/b is a preferred initiation site for population bursts occurring in the absence of fast GABAergic transmission. Sequential recruitment of neurons with different birthdates We next asked whether specific types of cells were activated at particular times of synchronization dynamics. A first series of experiments performed in GAD67-KI mice indicated that GABAergic neurons accounted for a significant fraction of EFNs at P7 (17±4%, n =6 movies, not shown). Interestingly, this suggests that GABAergic hub neurons are likely to be included in the EFN population. However, as fast GABAergic transmission is blocked, we did not explore further the involvement of these cells but focused on the differential involvement of glutamatergic neurons. We have recently shown that early-generated GABAergic neurons develop into functional hub cells [6] , suggesting that the network function of a cell could be partly predetermined by its embryonic origin. We, therefore, tested whether EGNs versus LGNs were differentially involved in network synchronization using inducible genetic fate mapping approaches. During development, pyramidal glutamatergic neurons transiently express the proneural bHLH transcription factor Neurogenin2 ( Ngn2 ) as they are becoming postmitotic. We have fate-mapped glutamatergic neuron precursors through the use of CreER, a tamoxifen-induced cre recombinase whose expression was placed under the control of the Ngn2 loci (that is, a Ngn2 CreERTM driver line [9] crossed with a Cre-dependent EGFP reporter line RCE:LoxP [10] ). Recombination of the reporter allele is achieved within 24 h upon administration of tamoxifen, therefore, temporally labelling glutamatergic cells as they become postmitotic. Temporal precision is due to the fact that Ngn2 expression is rapidly downregulated as soon as cells leave the cell cycle and start migrating [11] , [12] , [13] . Glutamatergic progenitors express Ngn2 in accordance with their exit from mitosis, hence the timing of Ngn2 in this population provides a precise proxy indicator of their birthdate [14] . By using the Ngn2 CreERTM driver and RCE:LoxP reporter lines and by providing tamoxifen at two separate embryonic time points (early E11–12 versus later ones E15–16), we were able to label temporally distinct populations of glutamatergic neurons (EGNs versus LGNs, see Methods ). The labelling thus obtained was quite sparse as 1–3 green fluorescent protein (GFP)-positive cells could be imaged in the same focal plane as the calcium movie at P7 ( n =24 GFP cells, 12 movies, Fig. 3b ). Immunohistochemical labelling for GFP at P15 and P60 revealed that EGNs and LGNs tended to localize in different regions. On average 2.5 EGNs and 7.2 LGNs were found in the CA3 region per section ( n =53 slices, Figs. 4 and 5 ). Interestingly, the layer distribution of GFP-positive cells in the neocortex matched the maturation gradient in this region as EGNs concentrated in deep layers while LGNs populated layers II/III ( Figs. 4a,c and 5a,c ). Similarly, different spatial distributions were observed in the hippocampus, with EGNs localized predominantly at the border with the stratum oriens , (53%, n =40 slices, 193 cells, Figs 4b and 5b ) while the majority of LGNs preferentially localized in superficial subregions of the stratum pyramidale (68%, n =13 slices, 187 cells, Figs 4d and 5d ). In addition, almost half of the hippocampal EGNs preferentially distributed in CA3a/b (49%) rather than CA3c (15%) or CA1 (7%, Fig. 4 ). Similar distribution patterns could be observed when comparing P15 and P60 ( Fig. 5e and Table 2). 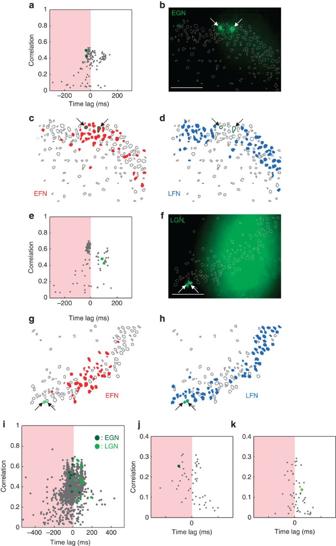Figure 3: Glutamatergic neurons are differentially recruited in synchronization build-ups according to their age. (a) Time-lag correlation graph plotting for each imaged neuron (grey points) the average correlation and average time of activation relative to all other cells for every network burst occurring, in the absence of fast GABAergic transmission, in the CA3 region of a P7Ngn2CreERTM;RCE:LoxPmouse hippocampal slice (tamoxifen treated at E12). Dark green circles indicate GFP-positive early-generated neurons (EGN). Note that they are both located in the EFN region (orange). (b) Photomicrograph of the region analysed in (a). Arrows indicate the two GFP-positive EGNs. Scale bar, 100 μm. (c,d) Contour map plotting the spatial distribution of imaged neurons. EFNs are red filled contours. GFPpositive EGNs are outlined in dark green. (d) Same as (c) for blue-filled LFNs. (e–h) Same as (a–d) but in a P7Ngn2CreERTM;RCE:LoxPmouse hippocampal slice (tamoxifen treated at E16). Light green circles indicate GFP-positive late generated neurons (LGN). (i) Pooled time correlation graph for all experiments in the absence of fast GABAergic transmission (n=12 movies). Dark green circles indicate EGNs while LGNs are marked in light green. (j) Same graph as (a) but in physiological conditions, recorded before the application of a GABAA-R antagonist. In this case, network synchronizations correspond to GDPs. The dark green circle marks the position of an EGN and indicates that this cell is firing at the GDP onset. (k) Same as (g) for a LGN neuron (light green) showing a late activation during GDPs. Figure 3: Glutamatergic neurons are differentially recruited in synchronization build-ups according to their age. ( a ) Time-lag correlation graph plotting for each imaged neuron (grey points) the average correlation and average time of activation relative to all other cells for every network burst occurring, in the absence of fast GABAergic transmission, in the CA3 region of a P7 Ngn2CreERTM;RCE:LoxP mouse hippocampal slice (tamoxifen treated at E12). Dark green circles indicate GFP-positive early-generated neurons (EGN). Note that they are both located in the EFN region (orange). ( b ) Photomicrograph of the region analysed in ( a ). Arrows indicate the two GFP-positive EGNs. Scale bar, 100 μm. ( c , d ) Contour map plotting the spatial distribution of imaged neurons. EFNs are red filled contours. GFPpositive EGNs are outlined in dark green. ( d ) Same as ( c ) for blue-filled LFNs. ( e – h ) Same as ( a – d ) but in a P7 Ngn2CreERTM;RCE:LoxP mouse hippocampal slice (tamoxifen treated at E16). Light green circles indicate GFP-positive late generated neurons (LGN). ( i ) Pooled time correlation graph for all experiments in the absence of fast GABAergic transmission ( n =12 movies). Dark green circles indicate EGNs while LGNs are marked in light green. ( j ) Same graph as ( a ) but in physiological conditions, recorded before the application of a GABAA-R antagonist. In this case, network synchronizations correspond to GDPs. The dark green circle marks the position of an EGN and indicates that this cell is firing at the GDP onset. ( k ) Same as ( g ) for a LGN neuron (light green) showing a late activation during GDPs. 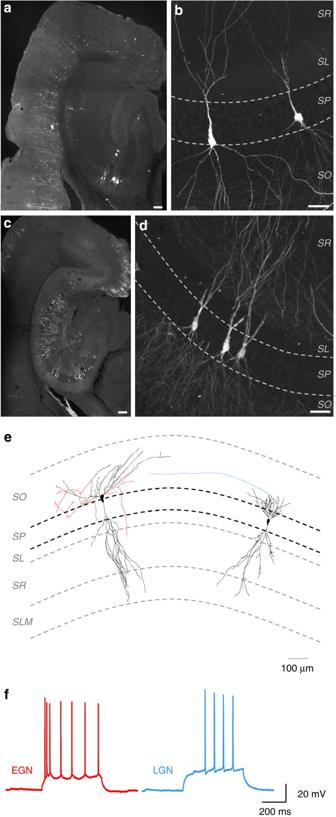Figure 4: Morpho-physiological properties of EGNs and LGNs in the hippocampus of adult and juvenile mice. Fate-mapped neurons are visible in the hippocampus and neocortex after GFP immunofluorescence detection inNgn2CreERTM;RCE:LoxPmouse slices. EGNs are relatively sparse in the hippocampus (a,b, tamoxifen gavage at E12) in comparison with LGNs (c,,dtamoxifen gavage at E15) throughout the CA1 and CA3 areas of the hippocampus. Early-generated pyramidal cells are preferentially localized in the deeper part of thestratum pyramidale(sp) of CA3a/b (a), while LGNs are distributed throughout the radial width of thestratum pyramidale(d). Note that EGNs populate the deeper layers of the neocortex (Cx) while LGNs are present in superficial layers. so:stratum oriens, sr:stratum radiatum, sl:stratum lucidum, slm:stratum lacunosum moleculare. Scale bars: 150 μm in a,c; 37.5 μm inb,d. (e) Neurobiotin-filled EGN (red) and LGN (blue), recorded in the CA3 region of P15–17 mice, and reconstructed with Neurolucida software. Neurons are placed on a schematic representation of the CA3 region. Axons are in colour, dendrites and soma in black. Note that the EGN is located closer to thestratum oriensthan the LFN. (f) EGN (red) and LGN (blue) firing responses to a positive current injection. Note that EGNs display a bursting firing pattern, whereas LGNs do not (e2). Full size image Figure 4: Morpho-physiological properties of EGNs and LGNs in the hippocampus of adult and juvenile mice. Fate-mapped neurons are visible in the hippocampus and neocortex after GFP immunofluorescence detection in Ngn2CreERTM ; RCE : LoxP mouse slices. EGNs are relatively sparse in the hippocampus ( a , b , tamoxifen gavage at E12) in comparison with LGNs ( c ,, d tamoxifen gavage at E15) throughout the CA1 and CA3 areas of the hippocampus. Early-generated pyramidal cells are preferentially localized in the deeper part of the stratum pyramidale (sp) of CA3a/b ( a ), while LGNs are distributed throughout the radial width of the stratum pyramidale ( d ). Note that EGNs populate the deeper layers of the neocortex (Cx) while LGNs are present in superficial layers. so: stratum oriens , sr: stratum radiatum , sl: stratum lucidum , slm: stratum lacunosum moleculare . Scale bars: 150 μm in a,c; 37.5 μm in b , d . ( e ) Neurobiotin-filled EGN (red) and LGN (blue), recorded in the CA3 region of P15–17 mice, and reconstructed with Neurolucida software. Neurons are placed on a schematic representation of the CA3 region. Axons are in colour, dendrites and soma in black. Note that the EGN is located closer to the stratum oriens than the LFN. ( f ) EGN (red) and LGN (blue) firing responses to a positive current injection. Note that EGNs display a bursting firing pattern, whereas LGNs do not (e2). 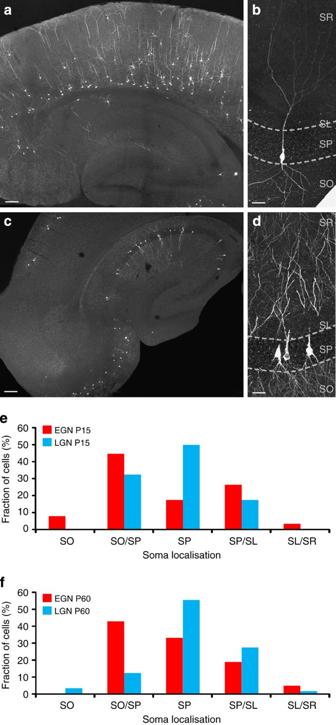Figure 5: The spatial distribution and morphological features of hippocampal EGNs/LGNs are similar at juvenile and adult stages. Fate-mapped neurons are visible in the hippocampus and neocortex after GFP immunofluorescence detection inNgn2CreERTM;RCE:LoxPmouse slices at P15. As at P60 (Fig. 4), EGNs are relatively sparse in the hippocampus (a,b, tamoxifen gavage at E12) in comparison with LGNs (c,d, tamoxifen gavage at E15) throughout the CA1 and CA3 areas of the hippocampus. Early-generated pyramidal cells are preferentially localized in the deeper part of thestratum pyramidale(sp) of CA3a/b (a), while LGNs are distributed throughout the radial width of thestratum pyramidale(d). Note that EGNs populate the deeper layers of the neocortex (Cx) while LGNs are present in superficial layers. so:stratum oriens, sr:stratum radiatum, sl:stratum lucidum. Scale bars: 150 μm ina,c; 37.5 μm inb,d. (e,f) Spatial distribution of the somata of EGNs (red, tamoxifen gavage at E12) and LGNs (blue, tamoxifen gavage at E15) along the radial axis of the CA3 hippocampal region measured at P15 (e) and P60 (f). Note that similar distributions are obtained at P15 and P60, with EGNs preferentially located at the border betweenstratum pyramidaleandstratum oriens(SO/SP) and LGNs located within thestratum pyramidale(SP). SO,stratum oriens, SO/SP, border betweenstratum pyramidaleandstratum oriens, SP,stratum pyramidale, SP/SL, border betweenstratum pyramidaleandstratum lucidum, SL/SR, border betweenstratum lucidumandstratum radiatum. Full size image Figure 5: The spatial distribution and morphological features of hippocampal EGNs/LGNs are similar at juvenile and adult stages. Fate-mapped neurons are visible in the hippocampus and neocortex after GFP immunofluorescence detection in Ngn2CreERTM;RCE:LoxP mouse slices at P15. As at P60 ( Fig. 4 ), EGNs are relatively sparse in the hippocampus ( a , b , tamoxifen gavage at E12) in comparison with LGNs ( c , d , tamoxifen gavage at E15) throughout the CA1 and CA3 areas of the hippocampus. Early-generated pyramidal cells are preferentially localized in the deeper part of the stratum pyramidale (sp) of CA3a/b ( a ), while LGNs are distributed throughout the radial width of the stratum pyramidale ( d ). Note that EGNs populate the deeper layers of the neocortex (Cx) while LGNs are present in superficial layers. so: stratum oriens , sr: stratum radiatum , sl: stratum lucidum . Scale bars: 150 μm in a , c ; 37.5 μm in b , d . ( e , f ) Spatial distribution of the somata of EGNs (red, tamoxifen gavage at E12) and LGNs (blue, tamoxifen gavage at E15) along the radial axis of the CA3 hippocampal region measured at P15 ( e ) and P60 ( f ). Note that similar distributions are obtained at P15 and P60, with EGNs preferentially located at the border between stratum pyramidale and stratum oriens (SO/SP) and LGNs located within the stratum pyramidale (SP). SO, stratum oriens , SO/SP, border between stratum pyramidale and stratum oriens , SP, stratum pyramidale , SP/SL, border between stratum pyramidale and stratum lucidum , SL/SR, border between stratum lucidum and stratum radiatum . Full size image We next compared the distribution of EGNs and LGNs in time correlation graphs obtained using calcium imaging at P7. We found that EGNs, in the presence of GABA A -R blockers, were activated during the build-up of network synchronization while the activation of LGNs occurred later ( Fig. 3 ). Indeed, GFP-positive cells in tamoxifen-induced Ngn2 CreERTM / RCE:LoxP pups at E11–12 ( n =10 GFP cells, five movies) or E15–16 ( n =14 GFP cells, seven movies) concentrated on the upper left side and upper right side of time correlation graphs, respectively, ( P <0.001, Fisher’s test, Fig. 3a–h ). This was clearly revealed by pooling the data from different slices ( n =10 GFP cells, five movies at E11–12, n =14 GFP cells, seven movies at E15–16, P <0.001, Fisher’s test, Fig. 3i ). EGNs were also activated at the onset of GDPs, while LGNs were activated later ( n =4, Fig. 3j ). We, therefore, conclude that at P7 EGNs form a sub-population of EFNs while LGNs are included in the LFNs group of cells. EGNs can trigger network bursts Given their early activation during synchronization, EGNs could be endowed with a specific network function in the absence of fast GABAergic transmission as early as P7. To test this hypothesis, we recorded in current-clamp conditions at P7, EFNs ( n =19 cells)/EGNs ( n =6 cells) or LFNs ( n =15 cells)/LGNs ( n =4 cells). Similarly to previous work [3] , [15] , we applied a phasic stimulation protocol, that is, short suprathreshold current pulses repeated at 0.05–0.2 Hz. Cell-network interaction was estimated based on the peristimulus time histogram plotting the occurrences of network bursts within a one second time window following cell stimulation [2] , [15] (see Methods ). A cell was considered as affecting network dynamics if the occurrences of network bursts in the first second following the stimulus was significantly different from chance level (see Methods and ref. 2 ). At P7, the stimulation of a single EFN rarely affected network dynamics: 3/19 EFNs significantly triggered network bursts ( P <0.05, see Methods ); for EFNs that induced a significant response, 12±1% of the phasic stimulations were followed by a network event within 1 s ( n =3, Fig. 6a ). As expected, LFNs neither impacted on network dynamics when stimulated: only 2/15 LFNs significantly triggered network bursts ( P <0.05, see Methods ) with 20±2.2% of stimulations followed by a network burst within 1 s, similarly to EFNs ( n =2, Fig. 6a ). In line with the above results, neither GFP-positive EGNs ( n =6) nor LGNs ( n =4) significantly affected the network dynamics when stimulated at P7 (not shown). 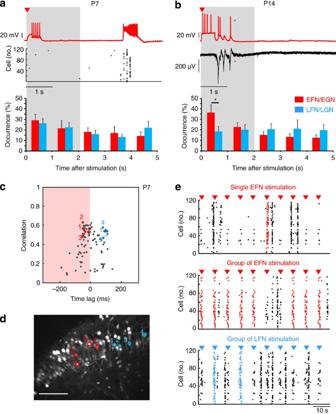Figure 6: EGNs can trigger synchrony as small assemblies at P7 and single-handedly at juvenile stages. (a,b) Simultaneous network and single-cell recordings of EFNs at P7 (a) and EGNs at P14 (b). Top Cells were recorded in current-clamp at resting membrane potential and stimulated with suprathreshold current injections (arrow head indicates stimulation). Middle Network activity was simultaneously recorded using calcium imaging at P7 (arasterplot of cell activation as a function of time), or extracellular electrodes at P4 (b). At P15 single-cell stimulation triggers network bursts (marked by *). Bottom: Pooled data histograms plotting the averaged distribution of network bursts within a 5 s time window following stimulation of a single EFN/EGN (red) or LFN/LGN (blue) (n=19 EFN/9 EGN,n=22 LFN/12 LGN). Asterisks mark time interval when the occurrence of network bursts is significantly different following the stimulation of single EGN or LGN (P<0.05, Studentt-test). Error bars are s.e.m. (c) Time correlation graph obtained from the analysis of a movie taken in the absence of fast GABAergic transmission in the CA3 region of a P7 mouse slice. Coloured points in the graph indicate the four-stimulated EFNs (red) and LFNs (blue). (d) Calcium fluorescence image of the recorded region. Outlined contours indicate the location of the four-stimulated EFNs (red) and LFNs (blue). Scale: 100 μm. (e) Rasterplots of cell activation as a function of time in the presence of bicuculline (10 μM) and 4-methoxy-7-nitroindolinyl-cagedL-glutamate (200 μM), during stimulation of one single EFN (top), during stimulation of the four EFNs (middle), and during stimulation of the four LFNs (bottom). The arrowheads indicate the times of light stimulation (10 stimulations in each case). Network bursts that were time-locked to light stimulations are highlighted in colour. Figure 6: EGNs can trigger synchrony as small assemblies at P7 and single-handedly at juvenile stages. ( a , b ) Simultaneous network and single-cell recordings of EFNs at P7 ( a ) and EGNs at P14 ( b ). Top Cells were recorded in current-clamp at resting membrane potential and stimulated with suprathreshold current injections (arrow head indicates stimulation). Middle Network activity was simultaneously recorded using calcium imaging at P7 ( a rasterplot of cell activation as a function of time), or extracellular electrodes at P4 ( b ). At P15 single-cell stimulation triggers network bursts (marked by *). Bottom: Pooled data histograms plotting the averaged distribution of network bursts within a 5 s time window following stimulation of a single EFN/EGN (red) or LFN/LGN (blue) ( n =19 EFN/9 EGN, n =22 LFN/12 LGN). Asterisks mark time interval when the occurrence of network bursts is significantly different following the stimulation of single EGN or LGN ( P <0.05, Student t -test). Error bars are s.e.m. ( c ) Time correlation graph obtained from the analysis of a movie taken in the absence of fast GABAergic transmission in the CA3 region of a P7 mouse slice. Coloured points in the graph indicate the four-stimulated EFNs (red) and LFNs (blue). ( d ) Calcium fluorescence image of the recorded region. Outlined contours indicate the location of the four-stimulated EFNs (red) and LFNs (blue). Scale: 100 μm. ( e ) Rasterplots of cell activation as a function of time in the presence of bicuculline (10 μM) and 4-methoxy-7-nitroindolinyl-caged L -glutamate (200 μM), during stimulation of one single EFN (top), during stimulation of the four EFNs (middle), and during stimulation of the four LFNs (bottom). The arrowheads indicate the times of light stimulation (10 stimulations in each case). Network bursts that were time-locked to light stimulations are highlighted in colour. Full size image Next, we hypothesized that the simultaneous activation of more than one EGN/EFN could be required to exceed a threshold frequency of synaptic or cellular activity that will lead to burst generation [4] . To test this, we simultaneously activated small groups of EFNs using targeted LASER (light amplification by stimulated emission of radiation) photostimulation to uncage 4-methoxy-7-nitroindolinyl-caged L -glutamate (200 μM). We compared multiple EFN versus LFN stimulations within the same slice. Neurons were targeted based on their time of activation during network synchronization rather than based on their developmental origin because too few GFP-positive EGNs can be simultaneously imaged within the same network. Confirming patch-clamp experiments, network bursts could not be reliably evoked by single EFN stimulation using glutamate uncaging ( Fig. 6c–e ). In contrast, multiple stimulations (three cells on average) of EFNs could more efficiently trigger network bursts than stimulating the same number of LFNs (bursts time-locked to the stimulation could be triggered in 41%±11% versus 24%±9% of the trials, n =10 slices, P <0.05, Student’s t -test or Mann–Whitney test, Fig. 6c–e ). In addition, we measured the probability of triggering a network burst as a function of the time elapsed from the last network event [3] . Notably, EFNs had a significantly higher stimulus effectiveness (see Methods ) compared with LFNs at any latency considered ( Supplementary Fig. S4 ). As expected, the lowest stimulus effectiveness was observed right after the occurrence of a network burst with values of 0.72±0.05 ( n =10) and 0.26±0.07 ( n =10) for EFNs and LFNs, respectively. We considered as network bursts neuronal coactivations whose peak amplitudes were significantly similar to those observed in control conditions (within three standard deviations from the average peak amplitude, P >0.01). However, we observed that photostimulation could also trigger local neuronal coactivations of smaller amplitudes in the spatial vicinity of stimulated cells ( Fig. 6e ); these were more reliably triggered by EFNs than LFNs (in 62%±9% versus 47%±10% of the trials, n =10 slices, P <0.001, Student’s t -test or Mann–Whitney test). Therefore, in the developing hippocampus (P7), the coactivation of EFNs assemblies can trigger network bursts, whereas single-cell stimulation is inefficient. The picture was different in juvenile mice as single-cell intracellular stimulation of more than half of EGNs (5/9 cells) significantly triggered network bursts within one second following the stimulation (with 40±12% of all stimulations followed by a network event, n =5, P <0.05, Fig. 6b , Methods ). In contrast, only 1/12 LGNs significantly triggered network events ( P <0.05, Methods ). Additionally, the fraction of network bursts occurring within the first second following stimulation relative to the total number of bursts within the first five seconds after stimulation, was significantly higher when EGNs were activated as compared with LGNs (37%±7% versus 19%±5% of network bursts occurred during the first second after stimulation, n =9 EGNs and 12 LGNs, P <0.05, Student’s t -test or Mann–Whitney test, see Methods , Fig. 6b ). We conclude that the threshold of excitation necessary for the generation of network bursts can be provided by a sub-population of early-generated and early firing glutamatergic neurons functioning as a small assembly in the developing hippocampus (P7) and gaining a single-cell triggering capacity after juvenile stages. EGNs form a morpho-physiologically distinct cell population We next asked whether EGNs constituted a morpho-physiologically distinct cell population. To this aim, we targeted for patch-clamp recordings EGNs ( n =12) and LGNs ( n =11) using GFP fluorescence in juvenile mice (P14 onwards). EGNs were morphologically distinct from LGNs. First, we found that the cell body of neurobiotin-filled EGNs was preferentially located at the border with the stratum oriens , whereas most LGNs distributed within stratum pyramidale and at the border with stratum lucidum ( Fig. 4e and Table 1 ). This is in agreement with the immunohistochemical data. Second, we observed that the first segment of the apical dendritic tree was significantly longer in EGNs than in LGNs ( P <0.05, Student’s t -test or Mann–Whitney test, Fig. 4e and Table 1 ). Last, EGNs differed from LGNs by their axonal collaterals, as 71% of EGNs ( n =12, Fig. 4e ) displayed axonal ramifications within several layers in contrast to 29% of LGNs ( n =11, Fig. 4e ). Regarding electrophysiological properties, we found that EGNs were more excitable than LGNs, as their resting membrane potential was closer to action potential threshold ( n =30 EGNs, and 32 LGNs, P <0.05, Student’s t -test or Mann–Whitney test, Table 1 ). Almost half of the EGNs (52%, n =30 EGNs) displayed bursts of spikes at the onset of short suprathreshold current pulses while significantly fewer LGNs were bursting (20%, n =32 LGNs, P <0.05, Fisher test, Table 1 , Fig. 4f ). Therefore, EGNs present specific morpho-physiological features in juvenile mice. Last, we asked whether these features remained into adulthood (P45–P120). As patch-clamp recordings from CA3 EGNs proved difficult in slices after P21, we first compared immunohistochemical labellings of EGNs and LGNs between P15 and P60. The distribution and dendritic properties of EGNs compared with LGNs remained significantly different at P60 ( Figs. 4 and 5 and Table 2 , P <0.05 Kolmogorov–Smirnov test). We also performed a few current-clamp recordings of EGNs at adult stages (P100–120, n =4) and found similar values for the propensity of burst firing, as well as resting or action potential threshold potentials as compared with juvenile stages ( P <0.05, Student’s t -test or Mann–Whitney test, Table 2 ). This indicates that the morpho-physiological differences we observed in juvenile stages persist into adulthood. Table 1 Comparison of the morpho-physiological properties of EGNs and LGNs at juvenile stages. Full size table Table 2 The basic properties of EGNs are not significantly different between juvenile and adult stages. Full size table We conclude that adult EGNs display distinct morpho-physiological properties that altogether should contribute to their higher propensity to fire at the onset of network synchronisation and to their function in triggering network bursts. We found a functional sub-population of CA3 pyramidal cells originating from the early stages of glutamatergic cell embryogenesis, enriched in the deeper parts of CA3a/b and endowed with distinct morpho-physiological properties. These findings confirm recent results suggesting functional heterogeneity of the principal cell population [17] and indicates that early embryonic origin is a common attribute of the previously described ‘pacemaker’ cell population [5] . These cells first operate as assemblies, in the developing hippocampus, and later become powerful single units capable of triggering network synchronization in the absence of fast GABAergic transmission. Therefore, the fact that ‘early-born’ cells are central nodes in the functional organization of hippocampal networks (ref. 6 and present work) may well be a general principle albeit with important differences between GABAergic and glutamatergic neurons, the former but not the latter exerting their roles at an early developmental stage [6] . We propose that the temporal origin of neurons is a critical determinant of single-cell function. Principal neurons are classically viewed as a fairly homogeneous cell population compared with their GABAergic partners. It is now well established that the heterogeneity of interneuron subtypes lies in their different spatio-temporal embryonic origins [18] . With some exceptions [16] , most cortical glutamatergic neurons share a common spatial origin, the ventricular zone of the pallium. However, we show here that the distinct temporal origin of EGNs confers them specific morpho-physiological features. It is now increasingly evident that principal cells display a high degree of genetic [19] , molecular [20] , [21] , morphological [22] , electrophysiological [23] and functional diversity [17] , [24] , [25] , [26] , [27] (see [28] for review). Interestingly, most of these properties segregate between deep and superficial pyramidal cell layers and most of the distinct features of EGNs had already been previously reported for hippocampal principal neurons. For example, bursting CA3 pyramidal cells were more frequently recorded at the border with stratum oriens and displayed a longer primary apical dendrite [29] , two properties that associated with EGNs. Our results show that single EGNs can synchronize neuronal activity when stimulated in the absence of fast GABAergic transmission starting from juvenile stages. Testing the network power of EGNs at late adult stages is unfortunately not feasible due to the irregularity of the network patterns occurring in the absence of fast GABAergic transmission after P45. How does this correlation between embryonic origin and network power operate? EGNs display specific intrinsic properties that make them likely to be efficiently activated at the onset of synchronization processes and to reliably activate other neurons. Thus, their resting membrane potential is closer to spike threshold and they tend to fire in bursts, a property having a primary role in reliable transmission of electrical signals [30] and frequently attributed to principal cells with a putative pacemaker function [5] , [31] , [32] . However, it is unlikely that a difference in intrinsic excitability has a determinant role on its own. Taken together, previous work, as well as present findings indicates that functional excitatory interactions may possibly be the most instructive parameter for the function of EGNs. In fact, it was shown that, in the absence of fast GABAergic transmission, hippocampal network bursts are initiated only when a threshold frequency of synaptic or cellular activity is exceeded [4] . Accordingly, the simultaneous activation of at least two EFNs reaches that threshold at immature stages, whereas stimulating one cell is sufficient at later time points, presumably when the density of connectivity is adequate. The selective ability of EFN/EGN cells to generate such significant activity rise is also likely to originate from their denser collateral innervation. Notably, EGNs are likely to form an interconnected network given that a ‘temporal matching rule’ was recently uncovered by which early populations of hippocampal principal cells have a higher chance to connect to each other [33] . Whether the presently described EGN population makes functional reciprocal connexions is difficult to address at present, given the low density of GFP-labelled cells per slice. It may also well be that related to their common origins, these cells display electrotonic interactions via gap junctions that would contribute to activity synchronization [34] . However, we do not have at present any evidence in favour of this hypothesis, even though similar cell types are more likely to be gap-junction connected. What would be the functional consequence of this regionalization of hippocampal principal layers into functionally and developmentally matched subnetworks? The CA3 region is a critical structure in the initiation and maintenance of several physiological network dynamics [35] . It was recently shown that neurons located in the deeper parts of the CA1 pyramidal layer were more likely to display place fields, as well as other features [17] . Within CA3, it is well documented that the CA3a/b subregions are particularly prone to the initiation of network events [37] , even though in some cases, network events can originate from CA3c [38] . Hence, EGNs may be selectively implicated in the generation of various physiological oscillations. Accordingly, we found here that EGNs were also early activated at the onset of GDPs, the physiological synapse-driven network oscillations occurring in the developing hippocampus during the first postnatal week [1] . Note that the challenge of GDPs relevance [39] has been infirmed recently [40] . Still, our previous study [2] clearly indicates that EGNs cannot single-handedly impact on GDP generation. The present finding may also be interpreted from the perspective of pathology because the network bursts generated when GABAergic signalling is blocked are traditionally considered to model epileptiform synchronization [5] , [41] , [42] , [43] . Yet, there is now good evidence that synchronised activities generated in these conditions bear only partial relevance to epilepsies. Indeed, epileptogenesis is always associated with considerable network remodelling, GABAergic transmission is not completely silent and sometimes even boosted [44] . Therefore, blockade of fast inhibition in naïve hippocampal slices is probably more relevant to the understanding of network synchronization per se . In any case, it will be interesting to test whether neurons will be differentially vulnerable to pathological insults according to their temporal origin [45] . If spared, given their higher firing propensity, EGNs could be activated at the onset of various epileptiform events, for example, during the recently described pre-ictal glutamatergic discharges emerging at the transition to seizure in slices from human epileptic patients [45] . In that case, small assemblies of EGNs could together preferentially participate in the expression of pathological activity patterns. Mice for inducible genetic fate mapping All animal use protocols were performed under the guidelines of the French National Ethic Comity for Sciences and Health report, in agreement with the European Community Directive 86/609/EEC. Double-homozygous Ngn2 CreER/CreER /RCE:LoxP +/+ (refs 9 , 47 ) male mice were crossed with 7- to 8-week-old wild-type Swiss females (C.E Janvier, France) for offspring production. To induce CreER activity, we administered a tamoxifen solution (Sigma, St Louis, MO) by gavaging pregnant mice as previously described [6] . Pregnant females crossed with Ngn2 CreER/CreER /RCE:LoxP +/+ males were force-fed at embryonic days 11–12 to 15–16 post vaginal plug in order to label Ngn2 -expressing precursors with GFP in the embryos. For simplification purposes GFP-expressing mice pups originating from these gavaged females are named tamoxifen-treated Ngn2 CreERTM ; RCE:LoxP . Only one-third of the pups of the gavaged females were positive for GFP. Slice preparation and calcium imaging Horizontal hippocampal slices were prepared from young (6–8-days-old that is, P6–8), juvenile (P14–20), or adult (P45–120) wild-type or tamoxifen-treated Ngn2 CreERTM ; RCE:LoxP ( n =150 slices) mouse pups with a Leica VT1200 S vibratome in ice-cold oxygenated modified artificial cerebrospinal fluid (ACSF) (0.5 mM CaCl 2 and 7 mM MgSO 4 ; NaCl replaced by an equimolar concentration of choline). Slices were 400 μm-thick to allow for the generation of network bursts after GABAA-R blockade with bicuculline or gabazine at P7 (refs 1 , 8 ), a time when many developing neurons still receive excitatory GABAergic inputs. In thinner slices, as previously reported [47] , bicuculline completely abolishes network activity ( Supplementary Fig. S2 , n =5). Slices were then transferred for rest (1 h) in oxygenated normal ACSF containing (in mM): 126 NaCl, 3.5 KCl, 1.2 NaH 2 PO 4 , 26 NaHCO 3 , 1.3 MgCl 2 , 2.0 CaCl 2 , and 10 D -glucose, pH 7.4. Fura2-AM-loading was obtained as described previously [2] . Imaging was performed with a multibeam multiphoton pulsed infrared LASER (Coherent) scanning system (LaVision Biotech) coupled to a microscope as previously described [49] . Images were acquired through a CCD (charge-coupled device) camera at a time resolution of 50–150 ms per frame. Slices were imaged using a X20, NA-0.95 or X10 NA-0.30 objective (Olympus). Patch-clamp recordings Sixty-five cells out of 111 were considered for the analysis of cell-network interactions as they offered stable recordings and good quality network recordings (with calcium imaging ( n =44) or field potential recordings ( n =21)). Intracellular solution was (in mM): 130 K-methylSO 4 , 5 KCl, 5 NaCl, 10 HEPES, 2.5 Mg-ATP, 0.3 GTP and 0.5% Neurobiotin. No correction for liquid junction potential was applied. Osmolarity was 265–275 mOsm, pH 7.3. Microelectrodes resistance was 4–9 MOhms. Uncompensated access resistance values below 20 MOhms were considered acceptable and results were discarded if they changed by >20%. excitatory postsynaptic potentials were analysed using the MiniAnalysis software (Synaptosoft, Decatur, CA). For stimulation experiments, the movie acquisition time was separated evenly between (1) a ~3 min resting period during which the cell potential was held close to Vrest (that is, zero current injection); (2) a ~3 min stimulation period during which phasic stimulation protocols were applied; (3) a ~3 min recovery period where the cell potential was brought back to resting membrane potential. Stimulation protocol: suprathreshold current pulses (15–200 pA, 500 ms) repeated at 0.1–0.2 Hz. The action potential threshold and amplitude, membrane capacitance and input resistance were measured offline using Clampfit. Vrest and Vthreshold were corrected for errors due to high input resistance values in developing neurons. Field potential recordings Extracellular field potentials were recorded with a multichannel DAM-8A amplifier (WPI) using glass electrodes filled with ACSF and placed in the stratum pyramidale. MEA recordings Extracellular field potentials and multiple unit activity were recorded using MEAs (MultiChannel Systems, Germany) comprising 60 electrodes in an ‘8 by 8’ arrangement (200 μm between electrodes). Signals were amplified ( × 1,200) and digitized at 10 kHz. Raw data was filtered (High Pass: 1 Hz, Band Stop: 50 Hz). Bursts of activity were detected as events above a 15-μV threshold. The rate of network bursts was computed using the MC_Rack built-in analyser. Matlab, Clampfit 10.1 (Axon Instruments, USA) and MiniAnalysis were used for analysis. Neurobiotin-filled cell recovering Slices were fixed overnight at 4 °C in Antigenfix, rinsed in PBS containing 0.3% Triton X-100 (PBST) and incubated overnight at room temperature in cy3-streptavidin (1/1,000 in PBST). Post-hoc analysis was performed using a confocal microscope (Zeiss LSM 510). Immunocytochemistry Animals (P15 and P60) were deeply anesthetized with a ketamine (50 mg ml −1 ) and xylazine (7.5 mg ml −1 ) solution at a dose of 2 ml kg −1 (i.p.) and perfused transcardially with 4% paraformaldehyde in PB (1 ml g −1 ). Horizontal brain sections (100 μm) were routinely processed for multiple immunofluorescence as described previously [6] . Morphometric analysis Fifty-four neurons were reconstructed with a computer assisted system attached to a microscope (Neurolucida, MicroBrightfield). Out of those, 41 were included in the morphometric analysis. Variables included: dendritic and axonal lengths, surfaces, number of terminals and of nodes (branching points where a process splits into two or more branches), soma size and length of the first segment of the primary apical dendrite. Nodes are selected manually. Cell and signal detection We used custom designed Matlab software [2] , [48] , which allowed: (1) automatic identification of loaded cells; (2) measuring the average fluorescence transients from each cell as a function of time; (3) detecting the onsets and offsets of calcium signals; (4) reconstructing the functional connectivity of the imaged network. For all the experiments included in the statistics, manual analysis was performed to correct for detection errors. Network synchronizations and cluster analysis Peaks of neuronal coactivations were detected as synchronous onsets peaks recruiting more neurons than expected by chance, as previously described [2] , [49] . To reveal if a characteristic pattern of cells was recruited in the build-up period of network synchronizations, we identified the cellular population activated in the 500 ms preceding the synchronous onsets peaks and converted it into a binary vector (1: cells activated/ 0: cells not activated). Given a total of m network synchronizations and n imaged active cells, a matrix of m rows and n columns was thus constructed. Similarity between rows, that is, cell populations, was measured using K-Means clustering, as previously described [2] . Briefly, we calculated the Hamming distance to identify a minimum of two clusters and cosine distance to quantify the similarity between vectors within a cluster, by using respectively ‘kmeans’ and ‘silhouette’ functions in Matlab. The average cosine distance within a cluster was used as a threshold parameter to establish the goodness of the clustering procedure and the consequent existence of characteristic cellular patterns. Clustering analysis on 20,000 reshuffled matrices was used to determine the thresholds with level of significance P <0.05. Surrogate data was generated by randomly reshuffling the population of cells activated in each network synchronization. Pairwise analysis and time-lag correlation graphs Pairwise analysis of the activation onsets time series of individual neurons was used to estimate the average correlation and average time of activation of each neuron relative to all others, as described in [2] . Given a calcium movie with a total of F frames and n active neurons, the firing of each neuron was converted into a binary time series of length F with unitary values corresponding to the firing onsets. The cross-correlation between the time series a and b of two neurons was calculated as follows: where σ a and σ b are the s.d. of the time series, t is the sampling time, T the movie duration and | τ |≤1 s. The maximum cross-correlation value and the time lag of its occurrence ( τ max ab ) were used to construct the correlation and time-lag matrices, CC max and τ max . The time-lag correlation graph was obtained by plotting for each neuron i its average values: . Cell-network interaction To establish whether the stimulation of a single or a group of neurons was able to trigger network synchronizations, we computed the peristimulus time histogram of the occurrence of network bursts [2] , [15] for the 5 s following the stimulus (1 s binning). A stimulation significantly triggered network bursts if the total number of events occurring within the first second after the stimulus was exceeding chance threshold with a level of significance P <0.05. Chance level was estimated when the cell was not stimulated [2] . The distribution of network bursts occurring in the 5 s following stimulation (1 s binning) was also quantified. We compared the values corresponding to the fraction of network bursts falling within the first 1 s bin after the stimulation of an EGN/EFN or LGN/LFN. Student t -test was used as these followed a normal distribution. The stimulus efficiency was calculated as the number of cells activated within the first second following the stimulation normalized to the average number of cells recruited in spontaneous network bursts. Photostimulation Experiments were performed using 200 μM of light-sensitive MNI-caged- L -glutamate (Tocris). Glutamate was uncaged at multiple spots in a given image (four maximum) using a 405-nm laser (exposure time: 10 ms, power: 4–6 mW/spot). The photostimulation path shared the same scanner with the infrared LASER, allowing for simultaneous calcium imaging and photostimulation. We did not observe any significant cross-talk between the excitation lights used for glutamate uncaging (405 nm) and calcium imaging (800 nm). How to cite this article: Marissal, T. et al . Pioneer glutamatergic cells develop into a morpho-functionally distinct population in the juvenile CA3 hippocampus. Nat. Commun. 3:1316 doi: 10.1038/ncomms2318 (2012).